Collagen-producing lung cell atlas identifies multiple subsets with distinct localization and relevance to fibrosis Collagen-producing cells maintain the complex architecture of the lung and drive pathologic scarring in pulmonary fibrosis. Here we perform single-cell RNA-sequencing to identify all collagen-producing cells in normal and fibrotic lungs. We characterize multiple collagen-producing subpopulations with distinct anatomical localizations in different compartments of murine lungs. One subpopulation, characterized by expression of Cthrc1 (collagen triple helix repeat containing 1), emerges in fibrotic lungs and expresses the highest levels of collagens. Single-cell RNA-sequencing of human lungs, including those from idiopathic pulmonary fibrosis and scleroderma patients, demonstrate similar heterogeneity and CTHRC1 -expressing fibroblasts present uniquely in fibrotic lungs. Immunostaining and in situ hybridization show that these cells are concentrated within fibroblastic foci. We purify collagen-producing subpopulations and find disease-relevant phenotypes of Cthrc1 -expressing fibroblasts in in vitro and adoptive transfer experiments. Our atlas of collagen-producing cells provides a roadmap for studying the roles of these unique populations in homeostasis and pathologic fibrosis. The lung is a complex organ with marked regional differences in structure and function. Important sub-structures in the lung include the conducting airways, responsible for filtering and delivering inhaled and exhaled air, the bronchovascular bundles, conduits for air, blood, and lymphatics, and the alveolar region, responsible for gas exchange [1] . Collagens play central roles in maintaining the organization and structural integrity of these distinct anatomic features [2] . Perturbation of collagen homeostasis is an important contributor to common lung diseases, including pulmonary fibrosis. However, the cells responsible for normal collagen production in each of these regions and for excess accumulation of collagen in fibrotic lung diseases have not been well characterized. It has been widely assumed that there is a single cell type, often called a myofibroblast and characterized by expression of the contractile protein alpha-smooth muscle actin (α-SMA), that is the major collagen-producing cell in the lung. However, previous work by ourselves and others suggest that α-SMA is an inconsistent marker of collagen-producing cells in in normal murine lungs and in murine models of pulmonary fibrosis [3] , [4] . To enhance progress in understanding the cellular and molecular mechanisms underlying normal collagen homeostasis and fibrotic lung diseases, a better understanding of the cells responsible for collagen production is urgently needed. The development of single-cell RNA-sequencing (scRNA-seq) allows us to evaluate the heterogeneity of tissue cell types with markedly improved precision. Several recently published studies have used this approach to characterize some of the mesenchymal populations in the lung. Zepp et al. identified mesenchymal alveolar niche cells and myogenic progenitor cells by using Axin2-CreER/Pdgfra-GFP/Wnt2-CreER reporter mice [5] . Xie et al. collected mesenchymal populations more broadly by sorting CD31, CD45, and Epcam-negative cells, and described 6–7 mesenchymal populations in normal and fibrotic murine lungs [6] . Another recent study performed scRNA-seq on all cells obtained with a single digestion protocol from fibrotic human lungs, but the overwhelming majority of cells obtained and analyzed were leukocytes and epithelial cells, with very few cells that were characterized as fibroblasts [7] . Overall, no studies to date have specifically focused on the cells responsible for production of collagen and other extracellular matrix (ECM) proteins and the anatomic location of these cell types in normal and fibrotic lungs. Here, we perform scRNA-seq of cells obtained with a protocol designed to capture all of the collagen-producing cells from normal and fibrotic mouse and human lungs. We use gene expression signatures to classify fibroblast subpopulations based on their anatomical localizations, and developed fluorescence-activated cell sorting (FACS) strategies to purify those populations. Through this approach, we identify molecularly distinct populations of fibroblasts that populate distinct anatomic locations, in the walls of conducting airways (peribronchial), surrounding bronchovascular bundles (adventitial) and embedded within the alveolar regions of the lung (alveolar). We also identify a unique population of Cthrc1 (collagen triple helix repeat containing 1) + fibroblasts, which are mostly found in fibrotic lungs in both mice and humans and expresses the highest levels of type 1 collagen and other ECM genes. Purified Cthrc1 + fibroblasts are more migratory than other subsets of collagen-producing cells and demonstrate an enhanced capacity to colonize the lungs of bleomycin-treated mice. These findings identify the distinct gene and cell surface protein expression patterns that characterize fibroblast subsets with distinct anatomic localizations. The Cthrc1 + subset we describe is likely to play an important role in the development of pulmonary fibrosis in mice and humans. scRNA-seq of murine lung cells in normal and fibrotic lungs We used Col1a1 -EGFP (Col-GFP) reporter mice to harvest all of the collagen-producing cells in murine lungs [8] . We induced lung fibrosis by intratracheally instilling bleomycin into two Col-GFP mice, and prepared a single cell suspension from the lungs 14 days after the bleomycin treatment. Two untreated Col-GFP mice were used as control. In addition to GFP + cells, we sorted GFP − cells to compare gene expression patterns in the cells responsible for collagen production to pattern seen in other cell types. We performed scRNA-seq of each sample using the 10x Genomics platform (Fig. 1a ). After quality filtering, we obtained 25953 cell profiles from all the GFP + and GFP − samples. We performed dimensionality reduction with canonical correlation analysis (CCA) subspace alignment and performed unsupervised clustering (Fig. 1b ) [9] . Analysis of representative markers identified clusters of endothelial, epithelial, and mesothelial cells as well as hematopoietic cells including macrophages, monocytes, neutrophils, dendritic cells, natural killer cells, and lymphocytes (Fig. 1c , Supplementary Fig. 1a ). To characterize the heterogeneity of collagen-producing cells in higher resolution, we focused on the cells from GFP + samples and removed all clusters with lineage markers, which did not consistently express Col1a1 except a small cluster of mesothelial cells (Fig. 1c ). Re-clustering of Col1a1 + cells revealed 12 clusters from 12,855 cells (Fig. 1d ). All the clusters included cells from both bleomycin-treated and untreated lungs except clusters 8 and 11, which were mostly from bleomycin-treated lungs (Fig. 1e , Supplementary Fig. 1b ). The clusters were categorized into two superclusters: one composed of clusters 0, 1, 2, 4, 6, 8, 10 with higher Col1a1 expression, and the other composed of clusters 3, 5, 7, 9 with higher Acta2 expression (Fig. 1f ). Cluster 11 is proliferating cells characterized by the expression of Mki67 and Cdc20 (Supplementary Fig. 1c ). Clusters 5 and 7 expressed smooth muscle cell markers such as Acta2 and Myh11 (Fig. 1f, g ). Cluster 9 expressed pericyte markers such as Mcam , Cspg4 and the highest level of Pdgfrb (Fig. 1g ). Fig. 1: scRNA-seq of murine lung cells in normal and fibrotic lungs. a Schematic of scRNA-seq sample preparation. b Uniform manifold approximation and projection (UMAP) plot of all cells colored by GFP + and GFP − samples. c Col1a1 expression on UMAP plot of all cells. See Supplementary Fig. 1a for identifying the lineages. NK, natural killer cell; Neut, neutrophil; Mac, macrophage; DC, dendritic cell; Mono, monocyte. d – f UMAP plots of Col1a1 + cells. d Unsupervised clustering identifies 12 clusters. e Cells from bleomycin-treated lung are shown in red. Cells from untreated lungs are shown in blue. f , g Gene expression levels for each gene. Full size image Identification of fibroblast subsets in normal lungs To further characterize these populations, we performed differentially expressed gene analysis and identified expression markers of clusters of interest (Fig. 2a ). Clusters 0, 1, 2, 10 shared common markers including Npnt and Ces1d (Fig. 2a ). Slc7a10 is specifically expressed in cluster 0 (Fig. 2a ). Clusters 4 and 6 shared some markers such as Pi16 and Dcn (Fig. 2a ). Cluster 4 uniquely expressed cytokines such as Il33 and Ccl11 , while cluster 6 uniquely expressed Adh7 (Fig. 2a ). Cluster 3 highly expressed Hhip , Aspn and Fgf18 (Fig. 2a ). Fig. 2: Identification of alveolar, adventitial, and peribronchial fibroblasts in untreated lungs. a Violin plots showing the expression levels in each cluster of representative marker genes. b , c Proximity ligation in situ hybridization (PLISH) images for Npnt (white) and Ces1d (magenta) ( b ), or for Pi16 (white) and Adh7 (magenta) ( c ). Magnified images of the white squares are shown in right panels. Arrows indicate co-localization of PLISH signals in GFP + cells. d PLISH images for Ccl11 (white) and Adh7 (magenta). e PLISH images for Hhip (white) and Aspn (magenta). Magnified images of the white square are shown in right panels. Arrows indicate co-localization of PLISH signals in GFP + cells. b – e Col-GFP is shown in green. DAPI signal is shown in blue. Scale bars, 50 μm. aw, airway; bv, blood vessel; cuff, cuff space. Images are representative of three experiments ( n ≥ 2). Full size image To examine the localization of these clusters in vivo, we used proximity ligation in situ hybridization (PLISH), a recently-reported in situ hybridization technology with high sensitivity and specificity [10] . The PLISH signal is observed as bright dots, which represent the cellular locations of target mRNA. In normal lungs, Col-GFP + cells were mainly detected at alveolar walls and adventitial cuffs surrounding large airways and arteries in bronchovascular bundles (Supplementary Fig. 2a ). We found that Col-GFP + cells in alveoli expressed both Npnt and Ces1d , markers for clusters 0, 1, 2, 10 (Fig. 2b ). We also detected Ces1d signals in airway epithelial cells, which is consistent with our whole lung scRNA-seq data (Supplementary Fig. 2b ), but not in Col-GFP + cells in bronchovascular cuffs (Fig. 2b ). Among these alveolar fibroblast clusters, cluster 0 was most prominent in the lungs of untreated mice (Fig. 1e , Supplementary Fig. 1b ). In contrast, Pi16 was expressed by Col-GFP + cells in the cuffs (Fig. 2c ). Adh7 , a marker for cluster 6, was also detected in Col-GFP + cells in the cuffs (Fig. 2c ). Furthermore, signals for Ccl11 were enriched in Col-GFP + cells in the cuffs (Fig. 2d ). These findings are consistent with a recent report, which identified Il33 -expressing stromal cells in the adventitial cuffs [11] , but also suggests that there is another kind of adventitial fibroblast characterized by Adh7 expression that does not express cytokine genes. A previous study identified Hhip + mesenchymal cells around airways in the lung [12] . PLISH for Hhip and Aspn , markers for cluster 3, also showed signal enrichment in subepithelial Col-GFP + cells around bronchi (Fig. 2e ). Those Hhip + Col-GFP + subepithelial cells were distinct from airway smooth muscle cells characterized by Actc1 expression (Supplementary Fig. 2c, d ). Three-dimensional imaging of cleared thick lung sections of Col-GFP mice revealed that those subepithelial Col-GFP + cells were intercalated between airway smooth muscle cells localized just below the airway epithelium (Fig. 3a, b , Supplementary Movie 1 ). Type 4 collagen staining showed that subepithelial Col-GFP + cells made contacts with epithelial basement membranes (Fig. 3c , Supplementary Movie 2 ). Adventitial fibroblasts closely associated with type 4 collagen surrounding the bronchovascular cuffs (Fig. 3c , Supplementary Movie 2 ). A previous report showed that Pdgfra + cells in alveolar walls have close association with type 2 alveolar epithelial cells (AEC2s) [13] . We crossed Col-GFP mice with Shh-Cre/Rosa26-lox-stop-lox-tdTomato mice, in which all epithelial cells in the lung express tdTomato [14] , to investigate the interaction of Col-GFP + cells and epithelial cells in alveoli. Consistent with the previous report, alveolar fibroblasts were located in close proximity to AEC2s (Fig. 3d , Supplementary Movie 3 ). Fig. 3: Characterization of alveolar, adventitial, and peribronchial fibroblasts. a – d Cleared thick sections of untreated lungs were imaged by confocal microscopy. Col-GFP is shown in green. DAPI is shown in blue. aw, airway; bv, blood vessel; cuff, cuff space. Images are representative from two experiments ( n ≥ 2). a , b α-SMA staining is shown in magenta. Arrows indicate peribronchial fibroblasts. a Magnified image of the white square is shown in the right panel. Scale bars, 50 μm (left panel), 20 μm (right panel). b Series of z-stack images were 3D-reconstructed. See also Supplementary Movie 1 . c Collagen 4 staining is shown in magenta. Magnified images of the white squares are shown in the right panels. Arrowheads indicate basement membranes. Scale bars, 50 μm (left panel), 20 μm (center and right panels). See also Supplementary Movie 2 . d Representative image of Shh-Cre/Rosa26-lox-stop-lox-tdTomato/Col-GFP mice. tdTomato signal is shown in magenta. Arrows indicate the close localization of alveolar fibroblasts and AEC2s. Scale bars, 50 μm. See also Supplementary Movie 3 . e Collagen-producing subpopulations identified are shown on UMAP plot of Col1a1 + cells. f Schematic showing the distinct localization of fibroblast subpopulations. Full size image These results identify 4 subclusters of alveolar fibroblasts (clusters 0, 1, 2, 10), two types of adventitial fibroblasts (clusters 4, 6), and a cluster of peribronchial fibroblasts (clusters 3) (Fig. 3e ). These fibroblast subpopulations have distinct localizations in different compartments of the lung (Fig. 3f ). Population comparison to previous studies Cluster 3 also expressed Lgr5 (Supplementary Fig. 3a ), suggesting that peribronchial fibroblasts may correspond to the Lgr5 + mesenchymal cells reported by Lee et al. [15] . Lgr6 was expressed by cluster 3 and some of the smooth muscle cells (Supplementary Fig. 3a ) [15] . Zepp et al. used Axin2 , Pdgfra , and Wnt2 to classify mesenchymal populations [5] . Axin2 was broadly expressed in all mesenchymal populations in our data set (Supplementary Fig. 3b ). Wnt2 was mainly expressed in clusters 0, 1, 2 (Supplementary Fig. 3b ). Sfrp4 and Wif1 were reported as markers for mesenchymal alveolar niche cells (MANC) [5] . Cluster 4 expressed Sfrp4 , and clusters 3, 6 expressed Wif1 in our data set (Supplementary Fig. 3b ). Clusters 5, 7, 9, which are smooth muscle cells and pericytes, expressed the markers of Axin2 + myofibrogenic progenitor (AMP), Notch3 and Gucy1a3 (Supplementary Fig. 3b ) [5] . Xie et al. reported Col13a1 and Col14a1 expressing fibroblasts [6] . Clusters 0, 1, 2 expressed Col13a1 , and clusters 4, 6 expressed Col14a1 (Supplementary Fig. 3c ). The population described as “myofibroblasts” in Xie et al. has the same markers as cluster 3, including Hhip and Aspn (Fig. 2a ). Higd1b and Cox4i2 , which are the markers of Pdgfrb hi populations in Xie et al., were expressed in pericytes (cluster 9), although we found pericytes from both untreated and bleomycin-treated lungs unlike Xie et al. (Fig. 1e , Supplementary Fig. 3c ) [6] . This apparent difference could be explained by differences in the digestion protocols used. The specific markers for the cells described as “lipofibroblasts” in Xie et al. such as Ear1 , Ear2, Mrc1 , or Clec4n , were all expressed in Ptprc (CD45) + Itgax (CD11c) + Siglecf + alveolar macrophages (Supplementary Fig. 1a , 3d ) [6] . General lipofibroblast markers such as Plin2 and Lpl were also expressed in clusters 0, 1, 2, consistent with previous reports that Pdgfra + Tcf21 + Col13a1 + alveolar fibroblasts have some phenotypic features of lipofibroblasts (Supplementary Fig. 3e ) [13] , [16] . Cthrc1 + cells express pathologic ECM genes in fibrotic lungs Next, we analyzed specific markers for cluster 8, which was mostly from bleomycin-treated lungs. Cluster 8 specifically expressed Cthrc1 , which was previously shown to be increased in bulk RNA sequencing from the lungs of patients with idiopathic pulmonary fibrosis (IPF) (Fig. 4a ) [17] . Other markers for cluster 8 include ECM-related genes such as Postn , Spp1 , Fn1, and Tnc (Fig. 4a ). Col1a1 and Col3a1 expression were also the highest in cluster 8 (Fig. 4a ). Feature plots of Col1a1 and Cthrc1 showed the correlation of the two genes in bleomycin-treated lungs (Fig. 4b ). Cthrc1 was specific for the population with the highest collagen expression and not significantly detected in other lung cells, while the myofibroblast marker, Acta2 was predominantly expressed by low collagen-expressing cells (Supplementary Fig. 4a ). PLISH for Cthrc1 and Col1a1 in bleomycin-treated lung sections showed that Cthrc1 was expressed at the periphery of clusters of Col1a1 + cells in the alveolar region (Fig. 4c ). To computationally investigate the potential progenitors of Cthrc1 + fibroblasts, we performed RNA velocity analysis, in which the direction of cellular differentiation is predicted based on the reads from both spliced and unspliced RNA [18] . Vectors pointing into cluster 8 mostly came from cluster 2, which expresses multiple markers of alveolar fibroblasts (Fig. 4d ). This analysis is consistent with the alveolar localization of Cthrc1 + fibroblasts. To further characterize the relevance of alveolar fibroblasts and cluster 8, we zoomed in on clusters 0, 1, 2, 8 (Fig. 4e ), and performed pseudotime trajectory analysis [19] . The resulting trajectory proposed a differentiation from cells in cluster 0 into clusters 1 and 2, with cells in cluster 8 forming a terminal state at the end (Fig. 4f ). These results suggest that Cthrc1 + fibroblasts are activated to produce pathologic ECM in fibrotic lesions and may principally differentiate from alveolar fibroblasts. Fig. 4: Cthrc1 + cells express pathologic ECM genes in fibrotic lungs. a Violin plots showing markers of cluster 8. b Expression levels of Col1a1 and Cthrc1 on UMAP plots. Cells from untreated lungs, bleomycin-treated lungs, or cluster 8 are shown separately in each column. c PLISH images for Cthrc1 (white) or Col1a1 (magenta) 14 days after bleomycin treatment. Col-GFP is shown in green. DAPI signal is shown in blue. H&E staining of serial section is also shown. Arrowheads indicate co-localization of Cthrc1 and Col1a1 in GFP + cells. Scale bar, 50 μm. Images are representative from three experiments ( n ≥ 2). d RNA velocity analysis overlaid on UMAP plot. Direction indicates transition towards the estimated future state of a cell. e UMAP plot showing only clusters 0, 1, 2, and 8. f Pseudotime trajectory analysis by Monocle 2. g Expression levels of Pdgfra and Col1a1 were analyzed along the pseudotime and fitted cubic smoothing spline curves are shown. The y -axis is scaled gene expression level. h Pdgfra and Col1a1 expression levels on UMAP plots. Full size image Interestingly, we found that the expression of alveolar fibroblast markers, such as Pdgfra , Npnt , Ces1d , and Tcf21 gradually decreased along the pseudotime towards cluster 8 (Fig. 4g, h , Supplementary Fig. 4b ), while ECM genes such as Col1a1 , Col3a1 , and Col5a1 gradually increased along the pseudotime (Fig. 4g, h , Supplementary Fig. 4b ). These results may indicate the differentiation of alveolar fibroblasts into functionally distinct ECM-producing cells. Peyser et al. suggested that activated fibroblasts were not uniquely defined from scRNA-seq of bleomycin-treated mouse lungs [20] . To clarify the discrepancy to our data, we analyzed their scRNA-seq data (GSE129605). After focusing on Col1a1 + cells, we found that a fraction of Col1a1 + cells, that expressed the highest levels of collagen and were mainly from bleomycin-treated lungs, grouped together and expressed cluster 8 markers such as Cthrc1, Tnc, Spp1 , and Fst , consistent with our findings (Supplementary Fig. 4c ). These pathologic fibroblasts were not bioinformatically identified as a distinct cluster possibly because there were relatively small number of Col1a1 + cells (~2000 cells) [21] . It is also possible that the dissociation conditions used in Peyser et al. did not capture all of these cells. scRNA-seq of normal and fibrotic lungs of human Next, we performed scRNA-seq of human lung cells to explore the heterogeneity of collagen-producing cells in normal and fibrotic lungs. We collected samples from explanted lungs of three IPF patients and two scleroderma patients, which allowed us to compare pathologic collagen-producing populations in two fibrotic diseases with different etiology. Three normal lung samples were collected from rejected lung transplant donors. We sorted lineage (CD31, CD45, CD235a, EPCAM) − cells to enrich mesenchymal cells. We also collected CD235a (erythrocyte marker) − cells as all lung cells. All the cell profiles were aggregated with mutual nearest neighbors (MNN) batch correction, which is effective for correcting diverse batch-to-batch differences (Fig. 5a ) [22] . We obtained 83316 cells after quality filtering. By analyzing representative markers, we identified T cells, B cells, dendritic cells, epithelial cells, endothelial cells, macrophages, and COL1A1 + mesenchymal cells (Fig. 5b , Supplementary Fig. 5a ). To characterize the heterogeneity of collagen-producing cell populations, we focused on lineage − samples and re-clustered COL1A1 + cells (Fig. 5c ). Unsupervised clustering identified 7 clusters from 48,587 cells (Fig. 5d ). Cell number of each cluster from each disease is shown in Supplementary Fig. 5b . Clusters 1, 3, 4 expressed PDGFRA , and clusters 0, 2, 6 expressed PDGFRB (Fig. 5e ). Cluster 0 expressed pericyte markers including RGS5 and MCAM , and clusters 2, 6 expressed the highest levels of smooth muscle markers including MYH11 and MYL9 (Fig. 5e ). We observed increased number of pericytes (cluster 0) both in IPF and scleroderma lungs (Supplementary Fig. 5b ). Cluster 1, which was enriched with cells from normal lungs, expressed alveolar fibroblast markers such as NPNT and CES1 (Fig. 5e , Supplementary Fig. 5b ). Cluster 4 expressed the markers of adventitial fibroblasts such as PI16 and DCN (Fig. 5e ). Cluster 5 markers include FGF18 and WIF1 , which were also expressed in peribronchial fibroblasts in mice (Fig. 5e ). Cluster 3 showed the highest COL1A1 expression and was enriched with cells from fibrosis patients (Fig. 5c, f , Supplementary Fig. 5b ). As seen in mice, CTHRC1 expression correlated with COL1A1 expression and was largely restricted to cells from fibrotic lungs, and ACTA2 expression was poorly correlated with COL1A1 (Fig. 5f ). These findings were consistent across all the samples we obtained (Supplementary Fig. 5c ). As we found in mice, CTHRC1 + cells also expressed other ECM genes such as TNC , POSTN , and COL3A1 (Fig. 5g ). Fig. 5: scRNA-seq identifies CTHRC1 + pathologic fibroblasts in human fibrotic lungs. a UMAP plot of all cells acquired by scRNA-seq of human samples. Cells were obtained from three normal lungs (green), three IPF lungs (red), and two scleroderma lungs (blue). b COL1A1 expression on UMAP plot. See Supplementary Fig. 5a for lineage identification. DC, dendritic cells; Mac, macrophage. c UMAP plot of COL1A1 + cells. d Unsupervised clustering identified 7 clusters. e Expression levels of representative genes are shown on UMAP plots. f Expression of COL1A1 , CTHRC1 , and ACTA2 are shown on UMAP plots. Cells from normal, IPF, and scleroderma lungs are shown separately in each column. g Expression levels of selected ECM genes on UMAP plots. Full size image To examine the consistency of our findings in larger data sets, we investigated scRNA-seq data from 29 normal and 32 IPF lungs [23] . After focusing on COL1A1 + cells, we found similar heterogeneous populations including RGS5 + CSPG4 + pericytes, MYH11 + MYL9 + smooth muscle cells, NPNT + CES1 + alveolar fibroblasts, and PI16 + DCN + adventitial fibroblasts (Supplementary Fig. 6a, b ). A fraction of cells, which were mainly from IPF lungs, highly expressed CTHRC1 and other ECM-related genes such as COL1A1 , COL3A1 , TNC , and POSTN (Supplementary Fig. 6c ). Emergence of CTHRC1 + fibroblasts in lungs of scleroderma patients was also reported in a recent scRNA-seq study [24] . Moreover, we analyzed scRNA-seq data (GSE128033) from Morse et al. [25] , in which the authors collected samples from 3 normal and 3 IPF lungs. We found that, consistent with our findings, a fraction of COL1A1 + cells expressed CTHRC1 and other ECM-related genes but not the highest level of ACTA2 (Supplementary Fig. 6d ). To localize pathologic fibroblasts in fibrotic lungs, we performed RNAScope in situ hybridization (ISH) and antibody staining for CTHRC1 in IPF lung sections (Fig. 6a ). The highest CTHRC1 RNA and protein expression was observed within fibroblastic foci, which are known as active sites of collagen production and leading edges of fibrogenesis (Fig. 6a ) [26] , [27] . These results support the idea that CTHRC1 + fibroblasts could contribute to pathologic fibrogenesis in IPF. Previous reports showed that fibroblastic foci in IPF are α-SMA-positive [26] . To investigate the relation between CTHRC1 + pathologic fibroblasts and α-SMA + cells, we stained sequential sections of IPF lungs for these markers (Fig. 6b ). Although fibroblastic foci populated with CTHRC1 + pathologic fibroblasts were also positive for α-SMA, α-SMA + cells were also evident outside fibroblastic foci (Fig. 6b ). Taken together with our scRNA-seq data showing the higher ACTA2 expression in smooth muscle cells and pericytes, these data suggest that α-SMA is not a specific marker of pathologic fibroblasts producing the highest levels of ECM. Fig. 6: CTHRC1 + pathologic fibroblasts are localized within fibroblastic foci in IPF. a Representative images of in situ hybridization (ISH) and immunohistochemistry (IHC) for CTHRC1 in the sections from three IPF patients. Scale bars, 100 μm. b CTHRC1 and α-SMA antibody staining in sequential sections of IPF lungs. Fibroblastic foci are outlined by dotted lines. Areas inside blue squares are magnified in lower panels. Arrows indicate α-SMA + cells outside CTHRC1 + areas. Images are representative from four IPF patients. Scale bars, 100 μm. Full size image FACS purification of fibroblast subsets One of the challenges in fibrosis research is a lack of methodology to purify mesenchymal subpopulations. To establish the methodology in mouse, we sought surface markers specific for each of the collagen-producing subpopulations. Pdgfra was widely expressed by alveolar and adventitial fibroblasts, although Cthrc1 + cluster 8 expressed relatively low levels of Pdgfra (Fig. 1g ). We found that adventitial but not alveolar fibroblasts expressed Ly6a (Fig. 7a ). Peribronchial fibroblasts were negative for Pdgfra but highly expressed Cd9 (Fig. 7a ). These results suggest that alveolar, adventitial, and peribronchial fibroblasts can be distinguished by the expressions of Pdgfra , Ly6a , and Cd9 , while smooth muscle cells and pericytes can be distinguished by Mcam (Fig. 7b ). To confirm this, we stained lung cells from untreated Col-GFP mice for these markers and performed sorting via FACS. After gating dump (CD31, CD45, EpCAM, Ter119) − and GFP + cells, we purified Mcam + cells, Mcam − Sca1 (Ly6a) + cells as adventitial fibroblasts, Mcam − Sca1 − Pdgfra + cells as alveolar fibroblasts, and Mcam − Sca1 − Pdgfra − CD9 + cells as peribronchial fibroblasts (Fig. 7c ). All GFP + cells were also sorted for comparison. We checked the expression of specific markers in sorted cells by quantitative Real Time PCR (qPCR) analysis. As expected, alveolar fibroblasts expressed Slc7a10 , Npnt , and Ces1d (Fig. 7d , Supplementary Fig. 7a ). Adventitial fibroblasts expressed Pi16 (Fig. 7d ). Il33 and Adh7 expressions were also enriched in adventitial fibroblasts, suggesting that the Sca1 + gating collected both clusters 4 and 6 (Supplementary Fig. 7a ). Peribronchial fibroblasts expressed Hhip and Aspn (Fig. 7d , Supplementary Fig. 7a ). Mcam + cells highly expressed Pdgfrb and Acta2 , which are the markers for pericytes and smooth muscle cells (Fig. 7d , Supplementary Fig. 7a ). These results suggest that alveolar, adventitial, peribronchial fibroblasts and Mcam + smooth muscle cells and pericytes can be purified based on Pdgfra, Sca1, and CD9 expressions in Col-GFP mice. Fig. 7: FACS purification of fibroblast subpopulations and their ability to colonize fibrosing lungs in adoptive transfer. a Expression levels of Ly6a and Cd9 on UMAP plots from murine data. b Violin plots showing expressions of surface markers on collagen-producing populations. c Gating strategy to purify Mcam + cells, adventitial fibroblasts, alveolar fibroblasts, and peribronchial fibroblasts from untreated lungs. d qPCR analysis of purified cells from untreated lungs. n = 5 mice. e Schematic for the adoptive transfer experiment. f The number of GFP + cells in host lungs were analyzed. n = 5 mice. g qPCR analysis of purified GFP + cells from the host lungs. Cells purified from untreated lungs were used as control. n = 5 mice. c , d , f , g Data are representative from two experiments. Source data are provided as a Source Data file. d , f , g Data are means ± SEM. Full size image A previous study showed that bulk GFP + cells from uninjured Col-GFP mice can colonize the lungs of bleomycin-treated, but not untreated mice after intratracheal adoptive transfer [28] . We used this transfer model to determine which of the subpopulations we identified have this capacity. We purified alveolar fibroblasts, adventitial fibroblasts, peribronchial fibroblasts, and Mcam + cells from untreated Col-GFP mice, and transferred identical numbers of each subpopulation into bleomycin-treated wild type mice (Fig. 7e ). Four days post-transfer, we harvested host lungs and counted GFP + cells via flow cytometry. Among the four populations, both adventitial fibroblasts and alveolar fibroblasts showed engraftment potential, with adventitial fibroblasts colonizing modestly better than alveolar fibroblasts (Fig. 7f ). The engraftment potential of peribronchial fibroblasts was about half that of alveolar fibroblasts (Fig. 7f ). Mcam + cells showed minimal engraftment potential, confirming our previously published results with Mcam + cells (Fig. 7f ) [28] . Although engraftment potential substantially varied among the populations, qPCR analysis of sorted GFP + cells from the host lungs showed that engrafted cells from all the groups upregulated Cthrc1 and Col1a1 compared to the untreated state (Fig. 7g , Supplementary Fig. 7b ), suggesting that these resting populations all have the potential to upregulate Cthrc1 and Col1a1 in response to local cues in the pro-fibrotic environment. To explore molecular mechanisms that might be responsible for the emergence of cluster 8 cells, we isolated alveolar fibroblasts from untreated Col-GFP mice and treated the cells with growth factors or cytokines including TGF-β, TNF-α, and EGF in vitro. We found that TGF-β stimulation induced several markers of cluster 8 cells, including Col1a1 , Cthrc1 , Postn , and Tnc , while TNF-α and EGF did not increase the expression of cluster 8 cell markers (Supplementary Fig. 7c ). Spp1 and Fst was not upregulated by TGF-β stimulation, suggesting that there are likely to be other factors in the fibrotic microenvironment involved in induction of the complete molecular phenotype of cluster 8 cells in vivo (Supplementary Fig. 7c ). Purified Cthrc1 + fibroblasts show pathologic phenotype Next, we developed methods to purify Cthrc1 + pathologic fibroblasts from bleomycin-treated mice. Time course analysis revealed that the expressions of cluster 8 markers, such as Cthrc1 , Fst , Spp1 and Col1a1 , peaked around day 10 after bleomycin treatment in Col-GFP + cells (Supplementary Fig. 8a ). In contrast, Pdgfra expression was downregulated after bleomycin treatment (Supplementary Fig. 8a ). Flow cytometry of bleomycin-treated Col-GFP mice showed the emergence of a Sca1 − Pdgfra − Col-GFP-high CD9-intermediate population not seen in untreated lungs (Fig. 8a ). We purified this population, which we refer to as cluster 8 here, and were also able to purify each of the collagen-producing populations from the lungs of bleomycin-treated mice (Fig. 8a ). qPCR analysis of purified cells showed that Cthrc1 expression was highly enriched in cluster 8 (Fig. 8b ). Consistent with our scRNA-seq data, Col1a1 expression was the highest in cluster 8 and Acta2 was enriched in Mcam + cells (Fig. 8b ). Of note, the markers for alveolar, adventitial, and peribronchial fibroblasts were similarly enriched by the same gating strategy used to purify the cells from untreated lungs (Supplementary Fig. 8b ). Fig. 8: Purified Cthrc1+ pathologic fibroblasts showed high migration and invasion capacity. a Gating strategy for purifying collagen-producing populations from bleomycin-treated lungs. b qPCR analysis of purified cells from bleomycin-treated lungs (day 10). n = 4 mice. c Representative images from gap migration assay with cells purified from bleomycin-treated lungs (day 10). Broken lines show initial cell-free zones. Col-GFP is shown in green. Scale bars, 500 μm. d Quantification of migration assay. n = 4 mice. *** p < 0.001, two-way analysis of variance followed by the Tukey–Kramer post-test. e The number of GFP + cells from the host lungs, which received purified cells from bleomycin-treated lungs, were analyzed. n = 5 (adventitial) or 6 (cluster 8 and alveolar) mice. ** p < 0.01, *** p < 0.001, one-way analysis of variance followed by the Tukey–Kramer post-test. f Whole lung imaging of host lungs. Col-GFP (donor cells) is shown in green. Autofluorescence in RFP channel is shown in white to visualize host lung cells. Images were maximum projection of z-stack images. Scale bars, 1 mm. b – f Data are representative from two experiments. b , d , e Data are means ± SEM. Source data are provided as a Source Data file. Full size image In fibrotic lungs, the cells that produce excess quantities of ECM are thought to arise in response to local injury and to migrate into injured areas where they form aggregates called fibroblastic foci that drive the fibrotic process [29] . We, therefore, sought to determine whether Cthrc1 + fibroblasts have increased the capacity to migrate in vitro and increased capacity to colonize the lungs of bleomycin-treated mice. We performed gap migration assays with cluster 8 cells, alveolar fibroblasts, and adventitial fibroblasts, which were purified from bleomycin-treated lungs on day 10 after treatment. Cluster 8 cells showed substantially higher migration capacity than alveolar or adventitial fibroblasts (Fig. 8c, d ). We also performed the intratracheal transfer of cluster 8 cells, alveolar fibroblasts, or adventitial fibroblasts purified from bleomycin-treated lungs. Two days after the transfer, cluster 8 cells showed markedly higher engraftment potential than either alveolar or adventitial fibroblasts (Fig. 8e ). Whole lung imaging of cleared host lungs also showed that transferred cluster 8 cells formed larger clusters in the host lungs than alveolar or adventitial fibroblasts (Fig. 8f ). These results suggest that, in addition to expressing higher levels of genes encoding ECM proteins, Cthrc1 + fibroblasts have high migratory capacity and are better able to colonize fibrosing lungs. Taken together, our results suggest that Cthrc1 + fibroblasts are pulmonary fibrosis-associated fibroblasts with a highly activated phenotype. Our scRNA-seq results provide the first systematic atlas of the molecular characteristics and anatomic locations of collagen-producing cells in the adult lung. Our results confirm that smooth muscle cells and pericytes express low levels of collagen in both mice and humans, but that there are unique populations of cells that express higher levels of collagen and reside in distinct anatomic locations—the walls of conducting airways, surrounding the bronchovascular bundles, and embedded within the gas-exchanging alveolar region. We speculate that each population plays unique functional roles in organizing and maintaining the unique structures of each of these regions and in fibrotic responses to regional insults. By comparing scRNA-seq results between normal and fibrotic lungs, we were also able to identify a unique population of cells that expressed the highest levels of collagens and other known components of the pathologic ECM, and were marked by high levels of expression of Cthrc1 in both mice and human. These cells were present within clusters of collagen-producing cells in fibrotic regions, and displayed marked increase in their capacity to migrate and to colonize the fibrosing lung after intratracheal transfer, suggesting that they play important roles in driving pulmonary fibrosis. In the absence of available lineage tracing mouse lines to definitively prove the origin of these cells, we used two different computational tools—RNA velocity and pseudotime trajectory analysis—which both suggested that these cells were most likely to have differentiated from a population of alveolar fibroblasts. Further support for this interpretation comes from our observations that levels of collagen expression progressively increased from populations of alveolar fibroblasts seen mainly in normal lungs, to populations of alveolar fibroblasts seen mainly in fibrotic lungs, to the Cthrc1 -expressing cells. In parallel, expression of several markers shared by normal alveolar fibroblasts, including Pdgfra , Tcf21 , and Npnt decreased progressively over this same continuum. Interestingly, both alveolar fibroblasts and adventitial fibroblasts purified from normal lungs and transferred back into the lungs of mice treated with intratracheal bleomycin were able to colonize the lungs of bleomycin-treated mice and markedly upregulated expression of Cthrc1 after transfer, suggesting substantial plasticity of these populations in response to a fibrotic in vivo environment. Myofibroblasts were first identified as contractile fibroblasts in granulation tissue [30] . After cutaneous injury, progenitor cells migrate into areas of injury and differentiate into myofibroblasts, which generate force and contract wounds [30] . An increase in the density of myofibroblasts in tissue is implicated in excessive collagen deposition in some disease settings [3] , [31] . In addition, adoptive transfer of purified fibroblasts in lung fibrosis showed upregulation of α-SMA together with ECM genes in transferred cells [28] , [32] . Our scRNA-seq data also show an increase in the number of Acta2 expressing cells in Cthrc1 + fibroblasts compared to their presumed progenitor, alveolar fibroblasts. However, the highest level of α-SMA expression is observed in smooth muscle cells and pericytes, which display low levels of collagen expression. These findings suggest that α-SMA is unsuitable as a specific marker of pathologic ECM-producing cells in the lung. We found that Cthrc1 is a marker for pathologic fibroblasts in pulmonary fibrosis. Cthrc1 is expressed in injured tissue and promotes cell migration [33] , [34] . Furthermore, invasive cancer cells express CTHRC1 and high CTHRC1 expression in tumors is associated with poor prognosis [35] , [36] . We found that Cthrc1 + fibroblasts from fibrotic lungs show high migration capacity and high potential to engraft when transferred into injured lungs. These findings are consistent with the previous suggestions that an invasive phenotype of fibroblasts promotes pulmonary fibrosis [37] , [38] , [39] , [40] . In humans with pulmonary fibrosis we and others have analyzed, CTHRC1 + fibroblasts emerged in pulmonary fibrosis associated with IPF and scleroderma, suggesting that there might be common mechanisms of fibrosis associated with CTHRC1 + fibroblasts in both diseases. Lee et al. and Zepp et al. reported mesenchymal cells similar to the peribronchial fibroblasts we describe here, that they reported can differentiate into smooth muscle cells after airway injury [5] , [15] . Although our scRNA-seq also showed some shared genetic signature between peribronchial fibroblasts and smooth muscle cells, lineage tracing experiments will need to be performed to determine whether these cells can serve as smooth muscle progenitors in vivo. Our RNA velocity analysis did not show vectors towards smooth muscle cells from peribronchial fibroblasts but this could be because the rate of differentiation is too slow in normal or bleomycin-treated lungs. Adventitial fibroblasts have been known to play important roles in tissue homeostasis and diseases [41] . Recent studies revealed IL-33-expressing stromal cells support the development of group 2 innate lymphoid cells (ILC2) and form niches for ILC2 in peripheral tissue [11] , [42] . In addition to these Il33 + adventitial fibroblasts, we revealed another kind of adventitial fibroblast characterized by Adh7 expression. The difference in physiological or pathological roles of these two adventitial fibroblasts is an intriguing question. Of note, we showed that adventitial fibroblasts have higher potential to engraft after transfer than alveolar fibroblasts. Taken together with a study showing Sca1 + stromal cells have stem cell-like phenotypes and are multipotent [43] , adventitial fibroblasts might also serve as progenitors for pathologic fibroblasts, perhaps in response to insults arising in proximal regions of the lung or insults arising from the lung vasculature. In conclusion, we have built an atlas of collagen-producing cells and identified several molecularly distinct cell types that occupy unique anatomic locations. We have also identified a novel population of cells unique to the fibrotic lung that produce the highest levels of collagens and other ECM proteins, and show the highest capacity to migrate and to colonize the fibrosing lung. The development of tools to mark, ablate and modify gene expression in each of these subtypes should provide important insights into the lineage relationships, homeostatic and pathologic roles of each of these cell types. Mice and bleomycin treatment Col-GFP mice were obtained from Dr. David Brenner at University of California, San Diego, CA, and maintained on the C57BL/6J background [8] . Shh-Cre (Stock No. 005622) and Rosa26-lox-stop-lox-tdTomato (Stock No. 007914) mice were obtained from the Jackson Laboratory. Although the Cre protein is fused with GFP in Shh-Cre mice, the expression of Shh is restricted to epithelial cells and Col-GFP + fibroblasts can be identified as GFP single-positive cells while epithelial cells are all tdTomato + in Col-GFP/Shh-Cre/Rosa26-lox-stop-lox-tdTomato mice. We obtained C57BL/6J mice from the Jackson Laboratory (stock no. 000664) as host mice for adoptive transfer experiments. Sex-matched mice between the ages of 8 and 12 weeks old were used for the experiments. Female mice were used for scRNA-seq. Both male and female mice were used in the other experiments. For fibrosis induction, mice were treated with 3 U/kg bleomycin in 70 μl saline by oropharyngeal aspiration, except host mice for transfer experiments, which were treated with 2 U/kg bleomycin. Mice were maintained in the UCSF specific pathogen-free animal facility in accordance with guidelines established by the Institutional Animal Care and Use Committee and Laboratory Animal Resource Center. All animal experiments were in accordance with protocols approved by the University of California, San Francisco Institutional Animal Care and Use Committee. Tissue dissociation Mouse lungs were harvested after perfusion through the right ventricle with 5 ml PBS. For human lungs, representative pieces were collected from whole lungs and cut into 5 × 5 × 5 mm pieces. Approximately 1 g tissue was randomly chosen from the pieces for digestion. After mincing with scissors, the tissue was suspended in protease solution [0.25% Collagenase A (Millipore Sigma), 1 U/ml Dispase II (Millipore Sigma), 2000 U/ml Dnase I (Millipore Sigma) in RPMI (Millipore Sigma) supplemented with 10 mM HEPES]. The suspension was incubated at 37 °C for 60 min with trituration by micropipette every 20 min. Then the cells were passed through 100 μm cell strainer (BD Biosciences), washed with PBS, and suspended in PBS with 0.5% bovine serum albumin (BSA) (Fisher BioReagents). Flow cytometry For scRNA-seq in mice, GFP + and GFP − cells were sorted after gating singlet, live (DAPI − ), and Ter119 − . For scRNA-seq in human, lineage negative (CD31, CD45, EPCAM, CD235a) − or all lung cells (CD235a − ) were sorted after gating singlet and live cells (DAPI − ). Donor cells for transfer experiments were sorted following magnetic negative selection for CD31, CD45, Epcam, and Ter119 by biotin-labeled antibodies and Dynabeads MyOne Streptavidin T1 (Thermo Fisher Scientific). The antibodies used were as follows: anti-CD9 (clone MZ3, PE; BioLegend), anti-CD31 (clone 390, biotin; BioLegend), anti-CD45 (30F-11, biotin; BioLegend), anti-Pdgfra (clone APA5, APC; BioLegend), anti-Mcam (clone ME-9F1, PerCP/Cy5.5; BioLegend), anti-Epcam (clone G8.8, biotin; BioLegend), anti-Sca1 (clone D7, PE/Cy7; BioLegend), streptavidin-APC/Cy7 (BioLegend), anti-hCD31 (clone WM59, PE/Cy7; BioLegend), anti-hCD45 (clone HI30, APC; BioLegend), anti-hEPCAM (clone 9C4, FITC; BioLegend), anti-hCD235a (clone HI264, APC/Cy7; BioLegend). Sorting was performed using FACS Aria III (BD Biosciences). Flow cytometry data were analyzed using the FlowJo v10. Human lung tissues The studies described in this paper were conducted according to the principles of the Declaration of Helsinki. Written informed consent was obtained from all subjects, and the study was approved by the University of California, San Francisco Institutional Review Board. Fibrotic lung tissues were obtained at the time of lung transplantation from patients with a diagnosis of usual interstitial pneumonia or scleroderma. Normal lung tissues were obtained from lungs rejected for transplantation by the Northern California Transplant Donor Network. scRNA-seq library preparation and sequencing We collected lung cells from two untreated and two bleomycin-treated (day 14) mice. After gating live cells and Ter119 − cells, GFP + and GFP − cells were sorted and each sample were processed separately. For human samples, lineage negative (CD31, CD45, CD235a, EPCAM) − cells or all lung cells (CD235a − ) were sorted. Approximately 1 × 10 5 cells were sorted for each sample. The sorted cells were re-suspended in PBS with 0.05% BSA and ~1 × 10 4 cells were loaded onto the Chromium controller (10x Genomics). Chromium Single Cell 3’ v2 reagents were used for library preparation according to the manufacturer’s protocol. For human samples, the libraries were stored at −20 °C and 2–3 batches were pooled for sequencing. The libraries were sequenced on Illumina HiSeq 4000 for mouse samples or NovaSeq 6000 for human samples. Sequencing data processing for mouse data Sequencing data were aligned to mouse genome mm10 with Cell Ranger version 2.0 (10x Genomics). The data were processed using the Seurat R package version 2.3.4 [44] . We excluded cells with fewer than 250 detected genes or larger than 10% percent mitochondria genes. Samples from untreated and bleomycin-treated lungs were aggregated with CCA subspace alignment [9] . For Col1a1 + cell analysis, we aggregated GFP + samples with CCA subspace alignment, and clusters which expressed lineage markers for hematopoietic, endothelial, epithelial, and mesothelial cells were removed. Col1a1 expression was not consistently detectable among each of these removed clusters except the small mesothelial cluster. Variable genes for dimensionality reduction were selected using FindVariableGenes function of Seurat. We performed graph-based clustering of the CCA reduced data using FindClusters function of Seurat (resolution = 0.6, dims.use = 1:20). Visualization of the clusters on a 2D map was performed with uniform manifold approximation and projection (UMAP) ( RunUMAP function of Seurat, dims.use = 1:20). Violin plots and UMAP plots overlaid with gene expression level were generated using Seurat. Differentially expressed genes of each cluster were identified using FindAllMarkers function of Seurat. RNA velocity and pseudotime trajectory analysis We used the velocyto R package v0.6 to estimate cell velocities from their spliced and unspliced mRNA content [18] . We generated annotated spliced and unspliced reads from the 10x BAM files via the dropEst pipeline, before calculating gene-relative velocity using kNN pooling with k = 25, fitting gene offsets using spanning reads and a gamma fit on the top/bottom 2% expression quantiles, and determining slope gamma with the entire range of cellular expression. We visualized aggregate velocity fields (using Gaussian smoothing on a regular grid) on the UMAP visualizations generated previously in Seurat. To generate cellular pseudotemporal trajectories we used the monocle R package v2.6.4 [19] . We ordered cells in an unsupervised manner (using genes with mean expression >1 and empirical dispersion ≥2*dispersion model estimate) and scaled the resulting pseudotime values between 0 and 1. Sequencing data processing for human data Sequencing data were aligned to human genome GRCh38 with Cell Ranger version 2.0 or 3.0. The data were first processed using the scran R package v1.10 22 . We excluded cells which were five median absolute deviation distant from the median value of library size, number of detected genes, or mitochondrial gene proportion. Variable genes were identified as genes with the largest biological components across all the samples following decomposition of the variance in expression for each gene into biological and technical components as described previously [45] . All samples were aggregated with MNN-batch correction [22] . Aggregated data and MNN dimensionality reduction were imported into Seurat. We performed graph-based clustering of the MNN reduced data using FindClusters function of Seurat (resolution = 0.3, dims.use = 1:19). For lineage sample analysis, clusters which expressed epithelial and endothelial markers were removed. Visualization of the clusters on a 2D map was performed with UMAP ( RunUMAP function of Seurat, dims.use = 1:19). Violin plots and UMAP plots overlaid with gene expression level were generated using Seurat. Differentially expressed genes of each cluster were identified using FindAllMarkers function of Seurat. Sequencing data processing for the large data set scRNA-seq data of IPF and normal human lungs from the IPF Cell Atlas preprint [23] . Following unsupervised clustering, stromal populations were identified on the basis of positive PDGFRB expression, resulting in a total of 6607 cells: 1144 control cells from 26 subjects and 5463 cells from 32 IPF patients. Gene expression was normalized by first scaling absolute UMI values to relative values of per 10,000 transcripts, followed by natural log transformation with a pseudocount of 1 (i.e., log((TPM/100)+1). Amongst the PDGFRB stromal cells, expressing was normalized with SCTransform 0.2.0 for the top 10,000 defined variable genes to regress out signals associated with the fraction of mitochondrial transcripts and the overall number of unique molecular identifiers (UMIs), using seed:7. Variable features were selected with Seurat 3.1.0 using the “mean variance plot” method, with a mean expression cutoff range between 0.15 and 4, and dispersion cutoff between 0.8 and 7. Amongst selected variable genes, only genes normalized by SCTransform were selected for PCA analysis under the default Seurat parameters. The top 6 dimensions were used for UMAP embedding with a neighborhood size of 20, a minimum distance of 0.1, for 1000 epochs. UMAPs featuring gene expression show the log((TPM/100)+1) values of expression per cell. Sequencing data processing for publicly available data sets Gene expression matrices of Peyser et al. (GSE129605) [20] and Morse et al. (GSE128033) [25] were processed using the Seurat R package version 2.3.4. Variable genes for dimensionality reduction were selected using FindVariableGenes function of Seurat. The samples were aggregated with RunMultiCCA function of Seurat. After performing graph-based clustering of the CCA reduced data using FindClusters function of Seurat, Col1a1 -expressing clusters were picked up for further analysis. UMAP plots overlaid with gene expression level were generated using Seurat. PLISH PLISH was performed as described previously with some modifications [10] . Lungs were fixed with 4% paraformaldehyde (PFA) for 6 h on ice and dehydrated with 30% sucrose overnight at 4 °C. Sixteen μm  sections were made from optimal cutting temperature compound (Sakura Finetek)-embedded frozen blocks. Target retrieval was performed by treating the sections with 10 mM citrate buffer containing 0.05% lithium dodecyl sulfate at 100 °C for 5 min and with 0.25 mg/ml pepsin in 0.1 M HCl at 37 °C for 5 min. The sections were incubated with H-probes in H-probe buffer at 37 °C for 2 h, followed by incubation with phosphorylated common bridge and circle oligonucleotides at 37 °C for 1 h. After incubation in ligation buffer at 37 °C for 2 h, the sections were incubated in RCA buffer at 37 °C overnight. Then the sections were incubated in labeling buffer containing Cy3 and Cy5-labeled oligonucleotide at 37 °C for 1 h. After washing with PBS with 0.05% tween 20, the sections were stained with chicken anti-GFP antibody (ab13970, Abcam) at room temperature for 1 h, followed by incubation with donkey anti-chicken alexa 488 secondary antibody (Jackson Immuno Research) and DAPI (Thermo Fisher) at room temperature for 1 h. The sections were mounted with ProLong Glass antifade Mountant (ThermoFisher). Images were taken using Zeiss 780 confocal microscope. 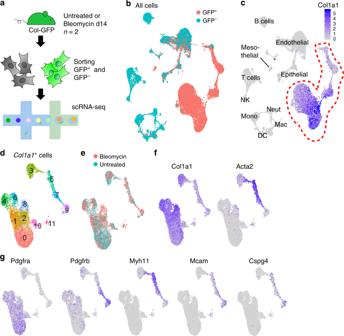Fig. 1: scRNA-seq of murine lung cells in normal and fibrotic lungs. aSchematic of scRNA-seq sample preparation.bUniform manifold approximation and projection (UMAP) plot of all cells colored by GFP+and GFP−samples.cCol1a1expression on UMAP plot of all cells. See Supplementary Fig.1afor identifying the lineages. NK, natural killer cell; Neut, neutrophil; Mac, macrophage; DC, dendritic cell; Mono, monocyte.d–fUMAP plots ofCol1a1+cells.dUnsupervised clustering identifies 12 clusters.eCells from bleomycin-treated lung are shown in red. Cells from untreated lungs are shown in blue.f,gGene expression levels for each gene. Oligonucleotide sequences used are listed in Supplementary Table 1 . Immunohistochemistry (IHC) and ISH staining for human samples Chromogenic IHC and in situ hybridization (ISH) staining for human samples were performed on an automated Bond RX immunostainer (Leica) as described below. 4 μm microtome sections of formalin-fixed, paraffin-embedded (FFPE) healthy and diseased IPF lung were collected on slides for IHC and ISH staining. For IHC staining, heat-induced epitope retrieval was performed by treating the sections with citrate buffer at 90 °C for 30 min. Sections were incubated with rabbit anti-CTHRC1 antibody (ab85739, Abcam) or anti-α-SMA antibody (ab5694, Abcam) at ambient temperature for 30 min, followed by Bond Polymer Refine Red Detection (DS9390, Leica). ISH staining was performed following Advanced Cell Diagnostic’s (ACD) standard Bond RX automated ISH protocol using RNAscope® 2.5 LS Reagent Kit-RED (Advanced Cell Diagnostics) and Bond Polymer Refine Red Detection (DS9390, Leica). RNAscope® LS 2.5 Probes against human CTHRC1 (413338, ACD) were ordered from ACD with hybridization optimized for human skin (EDTA for 15 min at 88 °C). Stained slides were digitized for image analysis using a Perkin Elmer P250 whole slide digital pathology slide scanner with 20×(IHC) or 40×(ISH) objective and extended focus scanning parameters. Imaging cleared lung tissues Untreated lungs of Col-GFP mice were fixed with 4% PFA overnight at 4 °C and then inflated with low-melting point agarose. 100 μm sections were made using a vibratome VT1000S (Leica). The sections were cleared using a CUBIC method as described previously [46] . After delipidation with Reagent-1A (10 wt% triton, 5 wt% NNNN-tetrakis (2-HP) ethylenediamine, 10 wt% urea, 25 mM NaCl), the sections were stained with anti-α-SMA-alexa 647 (R&D), or anti-collagen 4 (LSL) followed by donkey anti-rabbit IgG-alexa 647 (Thermo Fisher). The sections were then treated with refractive index-matching reagent (Reagent-2; 25 wt% urea, 50 wt% sucrose, 10 wt% triethanolamine) and imaged using W1 spinning disk confocal microscope (Nikon). Images were processed using Image J version 1.52i. 3D-reconstruction of z-stack images was performed using Icy version 2.0. For whole lung imaging after transfer, 4% PFA-fixed lungs were cleared with Reagent-1A and treated with Reagent-2, followed by imaging for GFP signal using Nikon AZ100 microscope configured as light sheet microscopy. Autofluorescence signal in RFP channel was used to visualize the lung structure. Maximum projection images were generated using Image J. Quantitative real-time PCR analysis Approximately 2000 cells were directly sorted into TRIzol reagent (Thermo Fisher), and RNA was isolated according to the manufacturer’s protocol. The RNA was reverse-transcribed using a Super Script IV VILO Master Mix with ezDNase Enzyme kit (Thermo Fisher). Quantitative Real-Time PCR was performed using 2x SYBR Green qPCR Master Mix (Bimake) with an ABI 7900HT (Applied Biosystems). 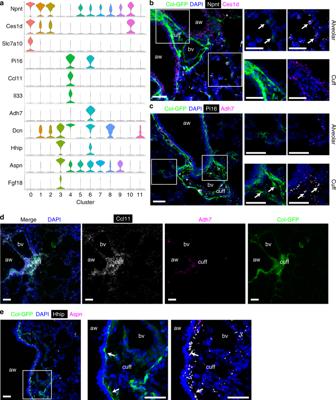Fig. 2: Identification of alveolar, adventitial, and peribronchial fibroblasts in untreated lungs. aViolin plots showing the expression levels in each cluster of representative marker genes.b,cProximity ligation in situ hybridization (PLISH) images forNpnt(white) andCes1d(magenta) (b), or forPi16(white) andAdh7(magenta) (c). Magnified images of the white squares are shown in right panels. Arrows indicate co-localization of PLISH signals in GFP+cells.dPLISH images forCcl11(white) and Adh7 (magenta).ePLISH images forHhip(white) andAspn(magenta). Magnified images of the white square are shown in right panels. Arrows indicate co-localization of PLISH signals in GFP+cells.b–eCol-GFP is shown in green. DAPI signal is shown in blue. Scale bars, 50 μm. aw, airway; bv, blood vessel; cuff, cuff space. Images are representative of three experiments (n≥ 2). Primer sequences are listed in Supplementary Table 2 . Primary alveolar fibroblast in vitro stimulation Alveolar fibroblasts were sorted from untreated Col-GFP mice. 1 × 10 5 cells were seeded into 48 well plates and cultured in DMEM (Corning) with 2% fetal bovine serum (FBS) (Gibco) and 1% penicillin–streptomycin (Gibco) for 24 h. Then medium was changed to serum-free DMEM with 1% penicillin/streptomycin for 24 h. After the serum starvation, medium was changed to serum-free DMEM with 1% penicillin/streptomycin, containing 1 ng/ml TGF-b (R&D), 10 ng/ml TNF-a (R&D), or 10 ng/ml EGF (Thermo Fisher). After 24 h stimulation, cells were lysed by directly adding 500 μl Trizol into the wells. Cell culture was performed under standard conditions (37 °C, 5% CO 2 ). Intratracheal adoptive transfer Donor cells were collected from untreated or bleomycin-treated (day 10) Col-GFP mice. 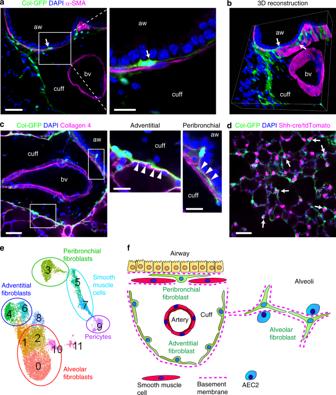Fig. 3: Characterization of alveolar, adventitial, and peribronchial fibroblasts. a–dCleared thick sections of untreated lungs were imaged by confocal microscopy. Col-GFP is shown in green. DAPI is shown in blue. aw, airway; bv, blood vessel; cuff, cuff space. Images are representative from two experiments (n≥ 2).a,bα-SMA staining is shown in magenta. Arrows indicate peribronchial fibroblasts.aMagnified image of the white square is shown in the right panel. Scale bars, 50 μm (left panel), 20 μm (right panel).bSeries of z-stack images were 3D-reconstructed. See also Supplementary Movie1.cCollagen 4 staining is shown in magenta. Magnified images of the white squares are shown in the right panels. Arrowheads indicate basement membranes. Scale bars, 50 μm (left panel), 20 μm (center and right panels). See also Supplementary Movie2.dRepresentative image of Shh-Cre/Rosa26-lox-stop-lox-tdTomato/Col-GFP mice. tdTomato signal is shown in magenta. Arrows indicate the close localization of alveolar fibroblasts and AEC2s. Scale bars, 50 μm. See also Supplementary Movie3.eCollagen-producing subpopulations identified are shown on UMAP plot ofCol1a1+cells.fSchematic showing the distinct localization of fibroblast subpopulations. Fibroblast subpopulations were sorted into PBS with 0.5% BSA. After resuspending the sorted cells in smaller volume of PBS with 0.5% BSA, live cell number was counted and cell concentrations were adjusted so that each sample had identical cell concentration. 70 μl of cell suspension was instilled into bleomycin-treated wild type mice (day 7) by oropharyngeal aspiration. 1–3 × 10 5 cells were transferred per mouse. Migration assay Fibroblast subpopulations were sorted into PBS with 0.5% BSA. 1 × 10 5 cells were resuspended in 100 μl DMEM (Millipore Sigma) with 2% fetal bovine serum (FBS) and dispensed into each well of Oris cell migration assay kit (fibronectin-coated) (Platypus Technologies). After 24 h incubation in a CO 2 incubator, the stoppers were removed and the wells were refilled with 100 μl DMEM with 2% FBS after washing with 100 μl PBS. The plate was incubated in a CO 2 incubator and GFP + cells were imaged after 24 and 48 hr using Zeiss spinning disk confocal microscopy. GFP + area in the central circle were quantified using Image J. Data analysis scRNA-seq data analysis was performed in R version 3.5.1. Statistical tests were performed in GraphPad Prism version 8.1.2. 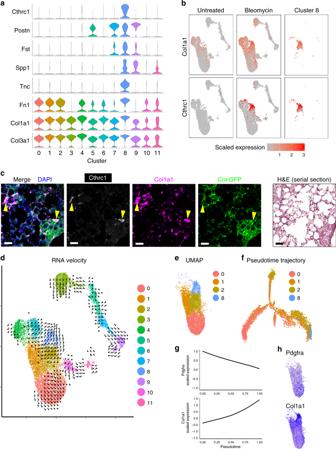Fig. 4: Cthrc1+cells express pathologic ECM genes in fibrotic lungs. aViolin plots showing markers of cluster 8.bExpression levels ofCol1a1andCthrc1on UMAP plots. Cells from untreated lungs, bleomycin-treated lungs, or cluster 8 are shown separately in each column.cPLISH images forCthrc1(white) orCol1a1(magenta) 14 days after bleomycin treatment. Col-GFP is shown in green. DAPI signal is shown in blue. H&E staining of serial section is also shown. Arrowheads indicate co-localization ofCthrc1andCol1a1in GFP+cells. Scale bar, 50 μm. Images are representative from three experiments (n≥ 2).dRNA velocity analysis overlaid on UMAP plot. Direction indicates transition towards the estimated future state of a cell.eUMAP plot showing only clusters 0, 1, 2, and 8.fPseudotime trajectory analysis by Monocle 2.gExpression levels ofPdgfraandCol1a1were analyzed along the pseudotime and fitted cubic smoothing spline curves are shown. They-axis is scaled gene expression level.hPdgfraandCol1a1expression levels on UMAP plots. 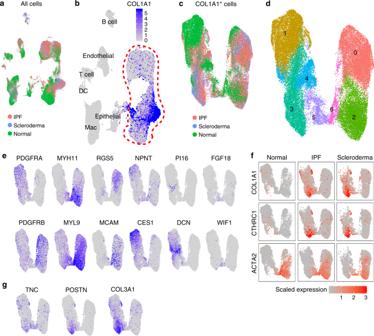Fig. 5: scRNA-seq identifies CTHRC1+pathologic fibroblasts in human fibrotic lungs. aUMAP plot of all cells acquired by scRNA-seq of human samples. Cells were obtained from three normal lungs (green), three IPF lungs (red), and two scleroderma lungs (blue).bCOL1A1expression on UMAP plot. See Supplementary Fig.5afor lineage identification. DC, dendritic cells; Mac, macrophage.cUMAP plot of COL1A1+cells.dUnsupervised clustering identified 7 clusters.eExpression levels of representative genes are shown on UMAP plots.fExpression ofCOL1A1,CTHRC1, andACTA2are shown on UMAP plots. Cells from normal, IPF, and scleroderma lungs are shown separately in each column.gExpression levels of selected ECM genes on UMAP plots. 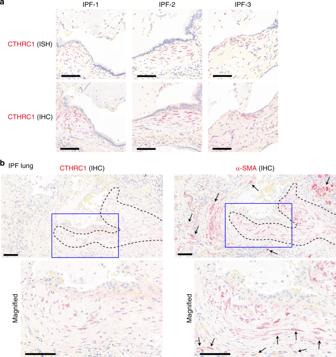Fig. 6: CTHRC1+pathologic fibroblasts are localized within fibroblastic foci in IPF. aRepresentative images of in situ hybridization (ISH) and immunohistochemistry (IHC) for CTHRC1 in the sections from three IPF patients. Scale bars, 100 μm.bCTHRC1 and α-SMA antibody staining in sequential sections of IPF lungs. Fibroblastic foci are outlined by dotted lines. Areas inside blue squares are magnified in lower panels. Arrows indicate α-SMA+cells outside CTHRC1+areas. Images are representative from four IPF patients. Scale bars, 100 μm. 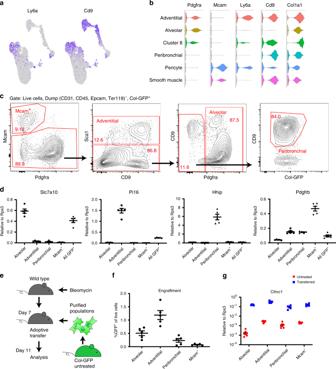Fig. 7: FACS purification of fibroblast subpopulations and their ability to colonize fibrosing lungs in adoptive transfer. aExpression levels ofLy6aandCd9on UMAP plots from murine data.bViolin plots showing expressions of surface markers on collagen-producing populations.cGating strategy to purify Mcam+cells, adventitial fibroblasts, alveolar fibroblasts, and peribronchial fibroblasts from untreated lungs.dqPCR analysis of purified cells from untreated lungs.n= 5 mice.eSchematic for the adoptive transfer experiment.fThe number of GFP+cells in host lungs were analyzed.n= 5 mice.gqPCR analysis of purified GFP+cells from the host lungs. Cells purified from untreated lungs were used as control.n= 5 mice.c,d,f,gData are representative from two experiments. Source data are provided as a Source Data file.d,f,gData are means ± SEM. 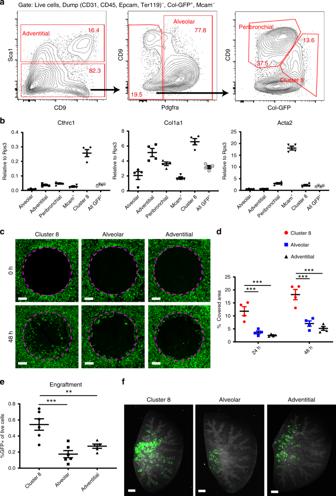Fig. 8: Purified Cthrc1+ pathologic fibroblasts showed high migration and invasion capacity. aGating strategy for purifying collagen-producing populations from bleomycin-treated lungs.bqPCR analysis of purified cells from bleomycin-treated lungs (day 10).n= 4 mice.cRepresentative images from gap migration assay with cells purified from bleomycin-treated lungs (day 10). Broken lines show initial cell-free zones. Col-GFP is shown in green. Scale bars, 500 μm.dQuantification of migration assay.n= 4 mice. ***p< 0.001, two-way analysis of variance followed by the Tukey–Kramer post-test.eThe number of GFP+cells from the host lungs, which received purified cells from bleomycin-treated lungs, were analyzed.n= 5 (adventitial) or 6 (cluster 8 and alveolar) mice. **p< 0.01, ***p< 0.001, one-way analysis of variance followed by the Tukey–Kramer post-test.fWhole lung imaging of host lungs. Col-GFP (donor cells) is shown in green. Autofluorescence in RFP channel is shown in white to visualize host lung cells. Images were maximum projection of z-stack images. Scale bars, 1 mm.b–fData are representative from two experiments.b,d,eData are means ± SEM. Source data are provided as a Source Data file. Reporting summary Further information on research design is available in the Nature Research Reporting Summary linked to this article.